A chemogenomic screening identifies CK2 as a target for pro-senescence therapy in PTEN-deficient tumours Enhancement of cellular senescence in tumours triggers a stable cell growth arrest and activation of an antitumour immune response that can be exploited for cancer therapy. Currently, there are only a limited number of targeted therapies that act by increasing senescence in cancers, but the majority of them are not selective and also target healthy cells. Here we developed a chemogenomic screening to identify compounds that enhance senescence in PTEN-deficient cells without affecting normal cells. By using this approach, we identified casein kinase 2 (CK2) as a pro-senescent target. Mechanistically, we show that Pten loss increases CK2 levels by activating STAT3. CK2 upregulation in Pten null tumours affects the stability of Pml, an essential regulator of senescence. However, CK2 inhibition stabilizes Pml levels enhancing senescence in Pten null tumours. Taken together, our screening strategy has identified a novel STAT3–CK2–PML network that can be targeted for pro-senescence therapy for cancer. Both genetic and epigenetic losses of the tumour suppressor gene PTEN are frequently observed in human cancers [1] . Interestingly, while monoallelic loss or mutation of PTEN drives cellular proliferation, complete inactivation of PTEN induces a senescence response, termed PTEN loss-induced cellular senescence (PICS) that opposes tumour development [1] . However, this response is not complete since upon Pten inactivation in vivo , a fraction of Pten null cells escapes senescence promoting tumor formation [1] , [2] . We have previously demonstrated that inhibition of either MDM2 or PTEN by means of small-molecule inhibitors enhances PICS thereby blocking tumour progression [1] . While this response depends on the functional activation of p53, recent findings demonstrate that senescence can also be activated in Pten ; Trp53 double null tumours by enhancing p27 levels through Skp2 inhibition [3] . These findings, together with the recent demonstration that senescent tumour cells activate an anti-tumour immune response [4] , have gained increasing interest for the clinical development of compounds that enhance senescence in cancer. However, the use of pro-senescence compounds in the clinic has been limited by their poor tolerability in cancer patients [3] . Indeed, the majority of these compounds block genes such as CDKs or MYC which are essential for the function of normal cells [3] . Identification of novel genes that regulate senescence in PTEN-deficient tumours without affecting normal cells would help to develop more effective and selective pro-senescence compounds for the treatment of different types of cancer [3] . This may be particularly relevant for prostate cancer therapy since PTEN-deficient prostate tumours conserve an intact p53 response even at late stage of tumorigenesis and may therefore benefit from treatments that enhance senescence by targeting p53 or its regulators. Here we report the results of a screening designed to identify ‘druggable’ targets regulating senescence in PTEN-deficient cells. Using chemogenomic and short hairpin RNA (shRNA) approaches, we found that the inhibition of CK2 enhances PICS without affecting normal cells. Our results demonstrate that CK2 is selectively upregulated in PTEN null cells and tumours and opposes PICS by affecting the stability of the promyelocytic leukaemia protein, PML, a known regulator of senescence in cancer [5] . Interestingly, our study also demonstrates that the upregulation of CK2 in Pten null tumours is mediated by activation of Stat3, which is highly phosphorylated in Pten null tumours. Taken together, our data provide new insight into the mechanisms that drive senescence evasion in tumour cells and validate the effectiveness of an integrated approach for the identification of ‘pro-senescence’ compounds in PTEN-deficient tumours. Identification of pro-senescence compounds For the identification of novel pro-senescence compounds that could be rapidly moved to the clinic, we took advantage of a drug library of 500 compounds including small-molecule inhibitors in advanced phase of preclinical development, or marked in the clinic for the therapy of cancer and additional disorders ( Supplementary Fig. 1a ). This library was created from a larger library of 90,000 compounds comprising: (1) New chemical entities, (2) compounds in advanced phase of development, (3) compounds already in the clinic for the treatment of cancer and different disorders. The rationale behind the selection of compounds in advanced phase of development was based on the fact that these compounds have already passed a significant number of tests both in vitro and in vivo (safety, toxicity and pharmacokinetics), thereby decreasing the risks of drug development failure due to adverse toxicity which is commonly observed in screenings based on new chemical entities [6] . Next, we set up a ‘pro-senescence’ screening platform, to evaluate the pro-senescence efficacy of these compounds in Pten −/− mouse embryonic fibroblasts (MEFs; Fig. 1a ). As previously reported, upon inactivation of Pten , 30% of the cells undergo senescence whereas the remaining 70% of Pten −/− cells bypass this arrest and continue to proliferate [7] ( Supplementary Methods ). This provides a screening window to identify compounds that enhance senescence by further decreasing proliferation of Pten −/− cells, as previously demonstrated for Nutlin-3, a MDM2 inhibitor [1] . Compounds that increased the percentage of senescent cells in the screening platform were designated as pro-senescence compounds based on two parameters: 1) inhibition of cell proliferation and 2) increase of SA-β-galactosidase staining (SA-β-gal), a prototypical senescence marker [1] ( Fig. 1a ). Experimentally, the screening was carried out in three steps. In the first step, 500 compounds were tested in triplicates using a single drug concentration (10 μM). Compounds that promoted a strong growth arrest in Pten null MEFs passed the first filter (efficacy filter; n =144/500). Positive hits were retested in triplicates in single concentration in both Pten fl/fl and Pten −/− MEFs to assess growth arrest in both cell types (specificity filter). Finally, the selective compounds ( n =33/144) were validated in duplicate in a concentration response assay (dose optimization filter). To perform IC50, data were normalized on each plate according to the negative control on Pten fl/fl and Pten −/− cells, respectively. IC50s were then evaluated on normalized data by using a four-parameter logistic model independently on each cell line. Twelve out of 33 compounds had a marked difference in the IC50 between Pten fl/fl and Pten −/− cells ( Pten −/− IC50 ≤ 60% Pten fl/flIC50 ) and were selected for the final step of the screening. Examples of compounds that did not pass the optimization filter despite a previous selectivity at single dosage were: Clotrimazole [8] , [9] , Clomipramine hydrochloride [10] , Nifedipine [11] , Trichostatin A [12] , [13] and Garcinol [14] (not specific cell growth arrest between Pten fl/fl and Pten −/− cells at the IC50). Finally, compounds were tested in SA-β-gal assay using both the cell lines to test for cellular senescence induction (SA-β–gal filter). Compounds that increased the SA-β-gal staining more than 30% as compared to dimethyl sulfoxide in Pten −/− cells passed this filter and were further validated by additional senescence markers (PAI-1 and p21) using RT–PCR and western blot. 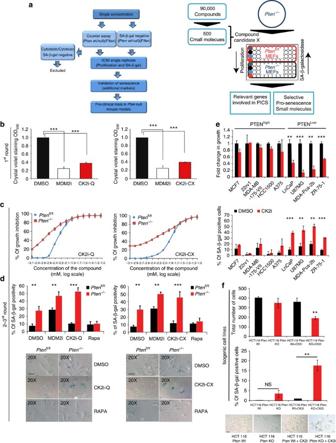Figure 1: Pro-senescence screening platform: CK2 drives senescence in PTEN-deficient cells. (a) Graphical representation of the pro-senescence screening cascade usingPtenfl/flandPten−/−primary MEFs (left panel). The assay is based on the assessment of cellular proliferation and senescence-associated SA-β-gal activity using compounds administered at single dose or in a dose–response assay (right panel). (b) Proliferation of primaryPten−/−MEFs treated with vehicle, the MDM2 inhibitor (MDM2i) Nutlin-3, the CK2 inhibitors quinalizarin (CK2i-Q) and CX-4945 (CK2i-CX) over a period of 5 days. (c) Dose–response assay in primaryPtenfl/flandPten−/−MEFs to determine the IC50 of CK2i-Q and CK2i-CX. (d) Quantification of SA-β-gal positivity inPtenfl/flandPten−/−MEFs treated with CK2i-Q, CK2i-CX, Nutlin-3 and Rapamycin (Rapa; upper Panel). Representative images of SA-β-gal staining in cells treated as indicated above (lower panel). Magnification is × 20. Scale bar, 10 μM (e) Proliferation and SA-β-gal positivity of different cancer cell lines treated with CK2i-Q. (f) Proliferation (upper panel), representative images and quantification of SA-β-gal positivity (lower panel) in HCT 116 isogenic cells treated with CK2i-Q. (c,d–f). Scale bar, 10 μM. Data are represented as mean±s.d.,n≥3. (***P<0.001, **P<0.01).Pvalue indicates that the statistical significance was measured by Student’st-test. Seven out of 12 compounds were found to have significantly enhanced senescence in Pten −/− cells as compared to the untreated control ( Supplementary Table 1a ). 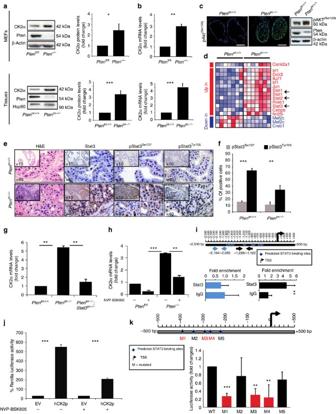Figure 2: CK2 transcription and protein levels are upregulated inPtenpc−/−tumour cells and STAT3 controls CK2 transcription. (a) Western blot analysis and quantification of CK2 and Pten protein levels in primaryPtenfl/flandPten−/−MEFs (upper panel) andPtenpc+/+normal prostates andPtenpc−/−prostate tumours (10–12weeks of age) (lower panel). (b) mRNA levels of CK2 in primaryPtenfl/flandPten−/−MEFs (upper panel) andPtenpc+/+normal prostates andPtenpc−/−prostate tumours (10–12weeks of age) (lower panel). (c) Immunofluorescence staining for pAKTSer129inPtenpc+/+andPtenpc−/−tumour sections. Western blot shows the protein level of Pten and pAKTSer129inPtenpc+/+normal prostates andPtenpc−/−prostate tumours (10–12weeks of age). Scale bar: 100 μM. (d) Heat map representation of the most upregulated and downregulated TFs predicted to bind to the CK2 promoter inPtenpc+/+normal prostates andPtenpc−/−prostate tumours (n=6). (e) IHC analysis of 12-week-old prostates fromPtenpc+/+andPtenpc−/−tumours, stained for total STAT3, pSTAT3Ser727and pSTAT3Tyr705. Magnification in all panels is × 40. Insets in all panels show the × 10 magnification Scale bar, 50 μM. (f) pSTAT3Ser727and pSTAT3Tyr705quantification of the experiment shown ine(n=4). (g) mRNA levels of CK2α in normal prostates and prostate tumours of the indicated genotypes. (h) Transcript levels of CK2α inPtenfl/flandPten−/−MEFs treated with or without the JAK2/STAT inhibitor, NVP-BSK805. (i) Schematic representation of the CK2α promoter region (upper panel) and the ChIP assay performed inPten−/−MEFs to confirm the Stat3 binding to the CK2α promoter (lower panel). Arrows indicate the length and position of the primers used in the experiment (j) Luciferase assay showing the promoter activity of human CK2α in cells treated with and without the JAK2/STAT inhibitor, NVP-BSK805. (k) Schematic representation of the mutated human STAT3-binding sites in the CK2 promoter region (upper panel) and luciferase activity (lower panel). Images (a,b,f,g,h,j,k) Data are represented as mean±s.d.,n≥3 (*P<0.05,**P<0.01, ***P<0.001).Pvalue indicates the statistical significance as measured by Student’st-test. Among these seven compounds, we found two bona fide (quinalizarin/CK2i-Q, CX-4945/CK2i-CX) [16] , [24] , [25] and one predicted (CK2i-S) [17] casein kinase 2 (CK2) small-molecule inhibitors, two cytotoxic compounds already available in the clinic (Carboplatin, Methotrexate [18] , [19] ), a KISS1 [20] , [21] and a DKK1 inhibitor (proprietary data of Sibi Spa; Supplementary Table 1a , Supplementary Table 2b and Supplementary Fig. 1b ). Examples of compounds that did not pass the SA-β–gal filter were: Penfluridol [22] and 5-Iodotubericidin [23] (did not induce cellular senescence in the SA-β-gal assay in both cell lines). Interestingly, bioinformatics analysis revealed that CK2 and DKK1 inhibitors targeted common genetic pathways, whereas Carboplatin, Methotrexate and KISS1 targeted distinct and independent pathways ( Supplementary Table 1b ). These compounds were also highly selective for Pten −/− cells (inhibition of proliferation for Pten fl/fl ≤20% and for Pten −/− ≥50%) as compared to a panel of anticancer compounds, already available in the clinic and included in the library ( Supplementary Fig. 1b,c ). Figure 1: Pro-senescence screening platform: CK2 drives senescence in PTEN-deficient cells. ( a ) Graphical representation of the pro-senescence screening cascade using Pten fl/fl and Pten −/− primary MEFs (left panel). The assay is based on the assessment of cellular proliferation and senescence-associated SA-β-gal activity using compounds administered at single dose or in a dose–response assay (right panel). ( b ) Proliferation of primary Pten −/− MEFs treated with vehicle, the MDM2 inhibitor (MDM2i) Nutlin-3, the CK2 inhibitors quinalizarin (CK2i-Q) and CX-4945 (CK2i-CX) over a period of 5 days. ( c ) Dose–response assay in primary Pten fl/fl and Pten −/− MEFs to determine the IC50 of CK2i-Q and CK2i-CX. ( d ) Quantification of SA-β-gal positivity in Pten fl/fl and Pten −/− MEFs treated with CK2i-Q, CK2i-CX, Nutlin-3 and Rapamycin (Rapa; upper Panel). Representative images of SA-β-gal staining in cells treated as indicated above (lower panel). Magnification is × 20. Scale bar, 10 μM ( e ) Proliferation and SA-β-gal positivity of different cancer cell lines treated with CK2i-Q. ( f ) Proliferation (upper panel), representative images and quantification of SA-β-gal positivity (lower panel) in HCT 116 isogenic cells treated with CK2i-Q. ( c , d – f ). Scale bar, 10 μM. Data are represented as mean±s.d., n ≥3. (*** P <0.001, ** P <0.01). P value indicates that the statistical significance was measured by Student’s t -test. Full size image A kinome shRNA screen validates CK2 as a pro-senescence target As an independent approach to validate the targets identified in the chemical screening, we employed ‘loss-of-representation’ or ‘drop-out’ genetic screens that allow the rapid screening of the effects of individual shRNAs in an shRNA library used to infect populations of Pten fl/fl and Pten −/− primary MEFs ( Supplementary Fig. 2a ). To this end, we obtained a lentiviral kinome knockdown library comprising 3,280 shRNAs targeting 672 mouse kinases. After infection of Pten fl/fl MEFs with the lentiviral library and Adeno-GFP or Adeno-Cre, PCR was used to isolate the integrated shRNAs from genomic DNA and deep sequencing of the shRNAs enabled the quantitative assessment of the relative abundance of these shRNAs in the cell populations before and after passaging of the cells ( Supplementary Fig. 2a ). We first filtered out shRNAs that were represented by less than 200 reads in the deep sequencing analyses of the early time points and then selected individual shRNAs whose representation in the shRNA population displayed little change or only modest changes in Pten fl/fl cells (less than an 8-fold change in representation at the late versus the early time point) but exhibited between 64- and 1,200-fold decreases in representation over time in the Pten −/− cells. A specific reduction in the representation of shRNAs over time in the Cre-infected cells was indicative of anti-proliferative or anti-survival effects of those knockdowns in the Pten −/− cells ( Supplementary Fig. 2b ). We conducted this screen twice and identified 75 shRNAs that fulfilled these criteria in both screens ( Supplementary Table 2a ). Consistent with the results of our chemical screen, among these hits was an shRNA targeting Csnk2a1 , which encodes CK2α, a subunit of CK2. Western blotting confirmed that CK2α was indeed downregulated in both Pten fl/fl and Pten −/− MEFs infected with the CK2 shRNA used in the screening ( Supplementary Fig. 2c ). Next we assessed senescence and found an increase in both, SA-β-gal staining and p53 protein levels using different CK2 shRNAs ( Supplementary Fig. 2d–f ). Additional hits included shRNAs targeting Akt2 and Akt3 , known downstream effectors of the PI3K pathway, and Plk1 , a gene previously shown to be essential for the viability of PTEN- deficient cells, suggesting that the screen was able to functionally identify genetic interaction partners in Pten mutant cells. However, these and additional targets were not identified by the chemical screening and were not tested for senescence induction in Pten null cells. CK2 inhibitors act as selective pro-senescence compounds CK2 inhibitors (CK2i) triggered a strong cell growth arrest selectively in Pten −/− MEFs with no detectable level of apoptosis at dosage below 30 μM. Inhibition of proliferation in cells treated with two CK2 inhibitors, quinalizarin [24] and CX-4945 (ref. 25 ) was similar to that of the cells treated with the MDM2 inhibitor, Nutlin-3, used as positive control [26] ( Fig. 1b ). Dose–response experiments performed with quinalizarin and CX-4945 and three additional CK2 inhibitors confirmed the high selectivity of these compounds for Pten −/− as compared to Pten fl/fl MEFs ( Fig. 1c and Supplementary Table 2b ). Moreover, CK2 inhibition by quinalizarin strongly increased SA-β-gal staining and both p21 and PAI-1 expression in Pten −/− as compared to Pten fl/fl cells ( Fig. 1d and Supplementary Fig. 3a,b ). 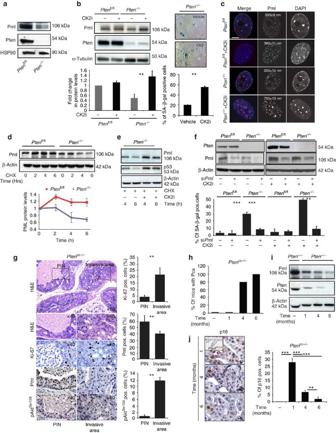Figure 3: CK2 inhibitors enhance senescence inPten−/−MEFs by controlling PML levels. (a) Western blot analysis of prostate tissues for Pml inPtenfl/flandPten−/−MEFs. (b) Western blot analysis for Pml protein levels (upper panel) and quantification (lower panel) inPtenfl/flandPten−/−MEFs before and after treatment with the CK2i-Q. Representative images and quantification of SA-β-gal positivity in MEFs treated with vehicle and CK2i-Q. (c) Immunofluorescence staining for Pml inPtenfl/flandPten−/−MEFs before and after treatment with the CK2i-Q. Quantification of the Pml bodies average size and s.d. is included in the panels. Scale bar, 5μM (d) Western blot analysis (upper panel) and quantification (lower panel) of Pml protein levels in primaryPtenfl/flandPten−/−MEFs after treatment with cycloheximide at different time points (0, 2, 4, 6 h) (e) Western blot analysis for PML and p53 in primaryPtenfl/flandPten−/−MEFs treated with both CK2i and cycloheximide at two different time points 4 and 6 h. (f) WB for Pml and Pten (upper panel) and SA-β-gal quantification forPtenfl/flandPten−/−MEFs transfected with a siPml and treated with the CK2i-Q. WBs have been run on two different gels (g) IHC staining and quantification for PML, Ki-67 and pAKTSer129in both PIN and invasive areas fromPtenpc−/−tumours at 15 weeks of age. Six samples per group were analysed. Invasive areas were defined using the following criteria: high percentage of Ki-67 staining and invasion of the stroma by the tumour epithelial cells. Scale bar, 50 μM (h) Percentage of mice affected with invasive prostate cancer inPtenpc−/−tumours at different stages (n=10). (i) Western blot analysis for Pml and Pten inPtenpc−/−tumours at different stages (1, 4 and 6 months).Ptenpc+/+normal prostate at 6 months is used as control (j) IHC staining (left panel) and quantification (right panel) of p16-positive cells inPtenpc−/−tumours at different stages (1, 4 and 6 months). Inset shows the negativity for p16 staining inPtenpc+/+normal prostate at 6 months. Scale bar: 50 μM. Images (b,e,f,g,h). Data are represented as mean±s.d.n≥3 (**P<0.01, ***P<0.001).Pvalue indicates the statistical significance as measured by Student’st-test. H&E, haematoxylin and eosin; Pos., positive. Next we checked whether this selectivity was also observed in human cancer cell lines expressing different PTEN levels ( Supplementary Table 3 ). Interestingly, CK2 inhibition resulted in an enhanced senescence response in PTEN-deficient cells when compared with human cancer cell lines expressing high levels of PTEN ( Fig. 1e ). These findings were also validated in a pair of HCT116 isogenic cancer cells with and without PTEN [27] ( Fig. 1f ). Finally, the selectivity of these compounds was tested in MEFs of different genetic backgrounds. Although CK2 inhibition induced a strong senescence response in Pten −/− cells, it did not selectively affect senescence in Trp53 −/− and H-Ras V12 infected MEFs ( Supplementary Fig. 3c,d ). Taken together, these data suggest that Pten −/− cells and PTEN-deficient human cancer cell lines are more sensitive than cells of other genetic backgrounds to CK2 inhibition. CK2 transcription and protein levels are controlled by STAT3 Next, we sought the mechanism underlying the selectivity of CK2 inhibitors for PTEN-deficient cells. CK2 is a serine/threonine protein kinase that functions as a tetramer of two α and two β subunits. The α subunits contain the catalytic activity, while the β subunits function as regulatory subunits, undergoing autophosphorylation [28] . Interestingly, while CK2 levels are consistently elevated in some subsets of human cancers, the mechanisms involved in CK2 upregulation remain unknown [29] . We detected a strong upregulation of CK2α protein (hereafter referred to as CK2) and mRNA levels in both Pten −/− cells and Pten null prostate conditional ( Pten pc−/− ) tumours but not in Pten fl/fl cells and Pten normal prostates ( Pten pc+/+ ), ( Fig. 2a,b and Supplementary Fig. 4a ). Of note, CK2 protein upregulation was also validated in PTEN −/− HCT116 human isogenic cancer cells ( Supplementary Fig. 4b ). The increased CK2 levels in Pten pc−/− tumours correlated with an increased CK2 kinase activity as demonstrated by phosphorylation of AKT (Ser129) , a specific marker of CK2 activity [30] ( Fig. 2c ). We next performed a bioinformatics analysis in Pten pc+/+ and Pten pc−/− tumours to identify transcription factors (TFs) responsible for CK2 mRNA upregulation. Towards this end, we analysed which of the most upregulated TFs in Pten pc−/− tumours could also bind the CK2 promoter and identified three different STAT family members as candidate TFs ( Fig. 2d ). In response to cytokines and growth factors, STAT proteins are phosphorylated by receptor-associated kinases and then form homo- or heterodimers that translocate to the nucleus, where they act as transcriptional activators [31] . Amongst these three STAT family members, signal transducer and activator of transcription 3, Stat3 was strongly phosphorylated at both Ser727 and Tyr705 in Pten pc−/− tumours as compared to the Pten pc+/+ normal prostates ( Fig. 2e,f ), whereas Stat1 and Stat2 were barely detectable by western blot analysis. Interestingly, Stat3 protein and mRNA levels were also strongly increased in Pten pc−/− tumours ( Fig. 2e and Supplementary Fig. 4c ). These data suggest that the activation of Stat3 in Pten pc−/− tumours may control CK2 transcription. To genetically validate this hypothesis, we intercrossed Pten lx/lx ; Pb Cre + mice with Stat3 lx/lx mice to generate Pten pc−/− ; Stat3 pc−/− mice. Inactivation of Stat3 in Pten pc−/− tumours ( Supplementary Fig. 4d,e ) decreased the mRNA levels of CK2 to the levels of the Pten pc+/+ normal tissue ( Fig. 2g ). CK2 mRNA levels were also strongly decreased in Pten −/− MEFs treated with NVP-BSK805, an inhibitor of the JAK2–STAT3 pathway [32] ( Fig. 2h ). To further validate the role of Stat3 in the regulation of CK2 transcription, we carried out a chromatin immunoprecipitation experiment in Pten −/− cells and detected a significant enrichment of Stat3 at the CK2 promoter in correspondence to a predicted STAT responsive element ( Fig. 2i ). As a positive control for this experiment, we used Socs3, a previously characterized STAT3 target gene [33] ( Supplementary Fig. 4f ). Experiments using a human CK2 promoter reporter confirmed that CK2 promoter activity was high in Pten −/− cells and that the inhibition of the Jak2/Stat3 pathway reduced CK2 promoter activity ( Fig. 2j ). Finally, we mutated five Stat3-predicted binding sites on the human CK2 promoter and we found that three out of the five mutants showed a profound reduction in the CK2 luciferase activity ( Fig. 2k ). In summary, these data demonstrate that Stat3 binds to the CK2 promoter and increases CK2 transcription in both Pten −/− cells and tumours. Figure 2: CK2 transcription and protein levels are upregulated in Pten pc−/− tumour cells and STAT3 controls CK2 transcription. ( a ) Western blot analysis and quantification of CK2 and Pten protein levels in primary Pten fl/fl and Pten −/− MEFs (upper panel) and Pten pc+/+ normal prostates and Pten pc −/− prostate tumours (10–12weeks of age) (lower panel). ( b ) mRNA levels of CK2 in primary Pten fl/fl and Pten −/− MEFs (upper panel) and Pten pc+/+ normal prostates and Pten pc −/− prostate tumours (10–12weeks of age) (lower panel). ( c ) Immunofluorescence staining for pAKT Ser129 in Pten pc+/+ and Pten pc −/− tumour sections. Western blot shows the protein level of Pten and pAKT Ser129 in Pten pc+/+ normal prostates and Pten pc −/− prostate tumours (10–12weeks of age). Scale bar: 100 μM. ( d ) Heat map representation of the most upregulated and downregulated TFs predicted to bind to the CK2 promoter in Pten pc+/+ normal prostates and Pten pc −/− prostate tumours ( n =6). ( e ) IHC analysis of 12-week-old prostates from Pten pc+/+ and Pten pc −/− tumours, stained for total STAT3, pSTAT3 Ser727 and pSTAT3 Tyr705 . Magnification in all panels is × 40. Insets in all panels show the × 10 magnification Scale bar, 50 μM. ( f ) pSTAT3 Ser727 and pSTAT3 Tyr705 quantification of the experiment shown in e ( n =4). ( g ) mRNA levels of CK2α in normal prostates and prostate tumours of the indicated genotypes. ( h ) Transcript levels of CK2α in Pten fl/fl and Pten −/− MEFs treated with or without the JAK2/STAT inhibitor, NVP-BSK805. ( i ) Schematic representation of the CK2α promoter region (upper panel) and the ChIP assay performed in Pten −/− MEFs to confirm the Stat3 binding to the CK2α promoter (lower panel). Arrows indicate the length and position of the primers used in the experiment ( j ) Luciferase assay showing the promoter activity of human CK2α in cells treated with and without the JAK2/STAT inhibitor, NVP-BSK805. ( k ) Schematic representation of the mutated human STAT3-binding sites in the CK2 promoter region (upper panel) and luciferase activity (lower panel). Images ( a , b , f , g , h , j , k ) Data are represented as mean±s.d., n ≥3 (* P <0.05,** P <0.01, *** P <0.001). P value indicates the statistical significance as measured by Student’s t -test. Full size image As PTEN is frequently lost in patients with prostate cancer, we checked the correlation between PTEN , CSNK2A1 and STAT3 mRNA levels in patients affected by advance prostate tumours by analysing two large microarray data sets. In the majority of invasive prostate cancers ( n =121), PTEN expression was significantly decreased as compared to the normal prostate samples ( n =72; Supplementary Fig. 5a,b ). These data reflect the high frequency of PTEN loss of heterozygosity in advanced prostate tumours. Interestingly, we found a correlation between decreased PTEN expression and increased STAT3 and CSNK2A1 mRNA levels in prostate cancer samples, in agreement with our findings in mouse tumours ( Supplementary Fig. 5a,b ). Moreover, CSNK2A1 overexpression and PTEN downregulation correlated with poor prognosis in patients affected by prostate cancer (both disease-free survival and overall survival; Supplementary Fig. 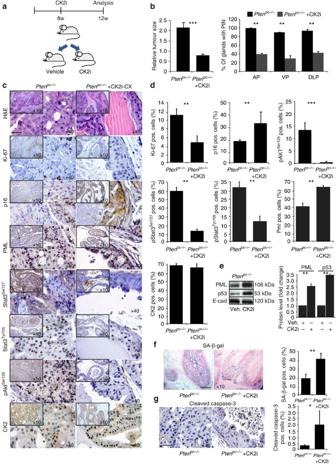Figure 4: The CK2 inhibitor, CX-4945, potentiates senescence by blocking tumour progression inPtenpc−/−mice. (a) Schedule of treatment used in the preclinical trial with the timing of the drug administration in thePtenpc−/−mice (n=12). (b) Quantification (left panel) of relative tumour size (APs) and percentage of PIN-affected glands in the anterior (AP), ventral (VP) and dorsolateral (DLPs) prostates ofPtenpc−/−mice in the two treatment groups. (c) Histopathological analysis ofPtenpc−/−prostate tumours before and after treatment with CK2i-CX and stained as indicated: H&E, Ki-67, p16, Pml, pAKTSer129, pStat3Tyr705, pStat3Ser727and CK2. Original magnification, × 40; insets show the × 10 magnification. Scale bar, 50 μM. (d) Quantification ofc. Sections from three mice were counted for each treatment group. (e) Representative western blot analysis for Pml and p53 protein levels inPtenpc−/−tumours treated with vehicle or CK2i-CX and quantification of protein levels. (f) SA-β-gal staining ofPtenpc−/−tumours from vehicle and CK2i-treated mice and the percentage of SA-β-gal positive cells is represented as a bar graph. (g) IHC staining and quantification of cleaved caspase-3 inPtenpc−/−tumours before and after treatment with CK2i-CX. Imaged (b,d,g) data are represented as mean±s.d.n≥3 (*P<0.05,**P<0.01, ***P<0.001).Pvalue indicates the statistical significance as measured by Student’st-test. H&E, haematoxylin and eosin; Pos., positive. 5c and Supplementary Table 4 ). Taken together, these data demonstrate that the upregulation of CSNK2A1 is a common feature of PTEN-deficient prostate tumours, emphasizing the need to target CK2 for cancer prevention and therapy in these tumours. CK2 inhibition enhances senescence by stabilizing Pml level We next sought to characterize the mechanism responsible for the increased senescence in Pten −/− MEFs upon CK2 inhibition. Recent evidence suggests that CK2 control the ubiquitin mediated degradation of PML, a known regulator of senescence in cancer [34] , [35] . Given the high CK2 levels in Pten −/− cells, we therefore checked Pml protein levels and found that Pml was decreased in Pten −/− cells as compared to the Pten fl/fl cells ( Fig. 3a and Supplementary Fig. 6a ). Interestingly, treatment of Pten −/− cells with quinalizarin [24] increased the protein levels of Pml, the SA-β-gal staining and enhanced the average size of Pml nuclear bodies ( Fig. 3b,c ). Next, we assessed Pml stability in Pten −/− MEFs and found that Pml half-life was significantly decreased as compared to the Pten fl/fl MEFs ( Fig. 3d ). However, inhibition of CK2 by quinalizarin increased the stability of Pml protein in Pten −/− cells treated with cycloheximide, restoring Pml and p53 levels ( Fig. 3e ). Note that under cycloheximide and quinalizarin treatment, the mRNA levels of Pml did not change ( Supplementary Fig. 6b ). Along this line, when Pten fl/fl and Pten −/− cells were treated with the proteasome inhibitor MG132, the protein levels of Pml increased, demonstrating that Pml is degraded through the proteasome as previously reported [34] ( Supplementary Fig. 6c ). Importantly, Pml knocked down by means of short interfering RNAs (siRNAs) blunted the senescence response in Pten −/− MEFs ( Fig. 3f ). Moreover, treatment with the CK2 inhibitor, quinalizarin, in cells transfected with different siPML failed to induce any pro-senescence effect in Pten null cells ( Fig. 3f and Supplementary Fig. 6e,f ). Figure 3: CK2 inhibitors enhance senescence in Pten −/− MEFs by controlling PML levels. ( a ) Western blot analysis of prostate tissues for Pml in Pten fl/fl and Pten −/− MEFs. ( b ) Western blot analysis for Pml protein levels (upper panel) and quantification (lower panel) in Pten fl/fl and Pten −/− MEFs before and after treatment with the CK2i-Q. Representative images and quantification of SA-β-gal positivity in MEFs treated with vehicle and CK2i-Q. ( c ) Immunofluorescence staining for Pml in Pten fl/fl and Pten −/− MEFs before and after treatment with the CK2i-Q. Quantification of the Pml bodies average size and s.d. is included in the panels. Scale bar, 5μM ( d ) Western blot analysis (upper panel) and quantification (lower panel) of Pml protein levels in primary Pten fl/fl and Pten −/− MEFs after treatment with cycloheximide at different time points (0, 2, 4, 6 h) ( e ) Western blot analysis for PML and p53 in primary Pten fl/fl and Pten −/− MEFs treated with both CK2i and cycloheximide at two different time points 4 and 6 h. ( f ) WB for Pml and Pten (upper panel) and SA-β-gal quantification for Pten fl/fl and Pten −/− MEFs transfected with a siPml and treated with the CK2i-Q. WBs have been run on two different gels ( g ) IHC staining and quantification for PML, Ki-67 and pAKT Ser129 in both PIN and invasive areas from Pten pc −/− tumours at 15 weeks of age. Six samples per group were analysed. Invasive areas were defined using the following criteria: high percentage of Ki-67 staining and invasion of the stroma by the tumour epithelial cells. Scale bar, 50 μM ( h ) Percentage of mice affected with invasive prostate cancer in Pten pc −/ − tumours at different stages ( n =10). ( i ) Western blot analysis for Pml and Pten in Pten pc −/ − tumours at different stages (1, 4 and 6 months). Pten pc+/+ normal prostate at 6 months is used as control ( j ) IHC staining (left panel) and quantification (right panel) of p16-positive cells in Pten pc −/ − tumours at different stages (1, 4 and 6 months). Inset shows the negativity for p16 staining in Pten pc+/+ normal prostate at 6 months. Scale bar: 50 μM. Images ( b , e , f , g , h ). Data are represented as mean±s.d. n ≥3 (** P <0.01, *** P <0.001). P value indicates the statistical significance as measured by Student’s t -test. H&E, haematoxylin and eosin; Pos., positive. Full size image Taken together, these data suggest that CK2 upregulation in Pten −/− cells favours the degradation of Pml, enabling a fraction of cells to bypass PICS. Consistently, CK2 inhibition potentiates senescence driven by Pten loss by stabilizing Pml protein levels. Finally, we checked the levels of PML and PTEN in a panel of prostate cancer cell lines and found a direct correlation between the level of PTEN and PML ( Supplementary Fig. 6g ). This was also associated with an increase in CSNK2A1 mRNA levels in PTEN-deficient cells ( Supplementary Fig. 6h ). We then checked in vivo whether CK2 upregulation in Pten pc −/− tumours could drive attenuation of senescence in vivo . During an early stage of tumorigenesis, Pten pc−/− tumours develop high-grade prostatic intraepithelial neoplasia, characterized by a strong senescence response. However, at late stage, Pten pc−/− tumours progress into more aggressive and invasive tumours [2] . We therefore monitored CK2 activity and Pml levels in Pten null tumours at the onset of tumour invasiveness (mice at 15 weeks of age). Immunohistochemistry (IHC) revealed that within the Pten pc−/− tumours the most invasive tumour glands were characterized by high CK2 activity (assessed by pAKT Ser129 ), high Ki-67 staining and low Pml protein levels, whereas the less aggressive glands displayed high levels of Pml and both low CK2 activity and Ki-67 positivity ( Fig. 3g ). A further time-course analysis in Pten pc−/− tumours at different stages, demonstrated that Pml levels progressively decreased during tumour progression ( Fig. 3h,i ). Moreover, decreased Pml levels correlated with a reduced percentage of p16-positive cells in the tumours and an increased tumour invasiveness ( Fig. 3j ). These data suggest that activation of CK2 in Pten pc−/− tumours drives a concomitant downregulation of Pml resulting in attenuation of senescence and promotion of tumour progression. Inhibition of CK2 enhances senescence in Pten pc−/− tumours We next evaluated in a preclinical trial in vivo , whether the inhibition of CK2 could block tumour progression in Pten pc −/− mice by stabilizing Pml protein levels and promoting senescence. To block CK2 in vivo , we used CX-4945, a novel CK2 inhibitor in clinical development [25] . CX-4945 was administered to Pten pc –/– mice at 8 weeks of age for 5 weeks ( Fig. 4a ). Interestingly, CX-4945 treatment decreased both tumour size and the number of PIN-affected glands in all the mouse prostate lobes analysed ( Fig. 4b ). This was associated with decreased staining of Ki-67, pStat3 Tyr705 , pStat3 Ser727 and increased p16 staining ( Fig. 4c,d ). Disappearance of pAKT Ser129 staining in Pten pc −/− tumours treated with CX-4945 was used as sign of impaired CK2 activity ( Fig. 4c,d ). Strikingly, Pml and p53 protein levels and SA-β-gal staining were also increased in Pten pc –/– tumours treated with CX-4945 ( Fig. 4e,f ). Finally, staining by caspase-3 revealed no major difference (0.5 versus 1.5% of positive cells per section) in apoptosis between the treatment groups, suggesting that the main function of CX-4945 in Pten pc –/– tumours is to enhance senescence rather than apoptosis ( Fig. 4g ). These findings substantiate the pro-senescence potential of CX-4945 in a genetically engineered mouse prostate model and identify a novel effective pro-senescence compound for prostate cancer therapy. Our findings also point to CK2-induced PML downregulation as a prominent mechanism of senescence attenuation and tumour progression in Pten null tumours. This is particularly noteworthy for human prostate cancer, where p53 function often remains functional even in advanced tumours, whereas PML levels are often found decreased [36] . Figure 4: The CK2 inhibitor, CX-4945, potentiates senescence by blocking tumour progression in Pten pc −/ − mice. ( a ) Schedule of treatment used in the preclinical trial with the timing of the drug administration in the Pten pc −/ − mice ( n =12). ( b ) Quantification (left panel) of relative tumour size (APs) and percentage of PIN-affected glands in the anterior (AP), ventral (VP) and dorsolateral (DLPs) prostates of Pten pc −/ − mice in the two treatment groups. ( c ) Histopathological analysis of Pten pc −/ − prostate tumours before and after treatment with CK2i-CX and stained as indicated: H&E, Ki-67, p16, Pml, pAKT Ser129 , pStat3 Tyr705 , pStat3 Ser727 and CK2. Original magnification, × 40; insets show the × 10 magnification. Scale bar, 50 μM. ( d ) Quantification of c . Sections from three mice were counted for each treatment group. ( e ) Representative western blot analysis for Pml and p53 protein levels in Pten pc −/ − tumours treated with vehicle or CK2i-CX and quantification of protein levels. ( f ) SA-β-gal staining of Pten pc −/ − tumours from vehicle and CK2i-treated mice and the percentage of SA-β-gal positive cells is represented as a bar graph. ( g ) IHC staining and quantification of cleaved caspase-3 in Pten pc −/ − tumours before and after treatment with CK2i-CX. Imaged ( b , d , g ) data are represented as mean±s.d. n ≥3 (* P <0.05,** P <0.01, *** P <0.001). P value indicates the statistical significance as measured by Student’s t -test. H&E, haematoxylin and eosin; Pos., positive. Full size image Since the first discovery that senescence could be enhanced in cancer cells, great effort has been made to identify novel pro-senescence compounds for cancer therapy. However, few small molecules have been identified so far that enhances senescence in tumours. Moreover, the majority of these molecules do not show selectivity for tumour cells and the risk of toxicity for cancer patients remains high. These targeted compounds include inhibitors of MDM2, MYC or CDK4, genes frequently deregulated in cancer, which also play a central role for the functional integrity of normal cells [3] . Senescence enhancement in normal cells may therefore increase the risk of organ toxicity in patients affected by cancer. Thus, identifying small-molecule inhibitors that increase senescence in cancer cells without affecting normal cells is an attractive strategy for cancer therapy. Senescence is a stable cell growth arrest which promotes tumour inhibition. Moreover, recent findings demonstrate that senescent tumour cells can be recognized and removed from cancerous tissues by components of both the adaptive and the innate immunity [37] , [38] . Indeed, senescent tumours cells are characterized by a senescence-associated secretory phenotype that can recruit and activate the tumour immune response [37] , [39] . Therefore, in stark contrast with current therapies (for example, chemotherapy) that mainly induce an apoptotic response, an effective pro-senescence therapy is expected to induce both a potent cell growth arrest and a specific antitumour immune response, thereby resulting in immune mediated tumour clearance. Here, we report the results of a screening strategy developed to identify pro-senescence compounds acting on a specific and relevant genetically defined subset of cancers, such as PTEN null tumours. The validity of this approach is supported by the effective identification of drug–genotype associations already established in previous preclinical models [26] , [40] , [41] and from the identification of CK2 inhibitors that show high selectivity in PTEN-deficient cells and tumours. Our screening approach coupling a small-molecule screening with a shRNA screen has allowed us to focus on a target that has been identified in both the screens, using complementary methodologies. Given that the tumour immune response is an essential component of the tumour suppressive function of senescence in cancer, these compounds could be tested in the clinic either alone or in combination with compounds that activate the tumour immune response or reprogramme the senescence-associated secretory phenotype as recently demonstrated from our group [7] , [42] . In this respect, we envisioned that our screening platform may also be implemented with different immune assays. For example, the conditioned media obtained from MEFs treated with selected pro-senescence compounds might be transferred on different immune cell subtypes to assess their immunostimulatory capabilities. Mechanistically, our findings have also identified a previously unknown STAT3–CK2–PML network that can be targeted to enhance senescence in cancer. While CK2 acts by promoting tumorigenesis in different settings, its role as senescence regulator in PTEN-deficient tumours remained elusive. It has been shown that CK2 controls proliferation and apoptosis by promoting the phosphorylation of several proteins including p53 (ref. 43 ). Intriguingly, although CK2 is upregulated in several cancers, the mechanism underlying such upregulation was ambiguous. In this respect, our findings demonstrate that activity of the JAK/STAT3 pathway, one of the most commonly deregulated pathways in cancer, resulted in CK2 overexpression, thus providing one of the mechanisms by which CK2 level is increased in cancer. Another intriguing finding of this study is the discovery that Pten null tumours at the late stage of tumorigenesis exhibit decreased levels of the tumour suppressor Pml, an essential regulator of oncogene induced senescence [5] . Previous evidence demonstrates that the Pten pc−/− mice develop senescence in tumours at an early stage; however, the majority of these tumours eventually progress to invasive prostate cancer bypassing the initial senescence response driven by Pten loss. Our time-course analysis in Pten null tumours analysed at different stages demonstrates that Pml levels decrease during tumour progression in parallel with p16 staining positivity a marker of senescence. Importantly, we also detected increased levels of pAKT Ser129 staining, a marker of CK2 kinase activation in tumour regions with low level of Pml. This is consistent with a model in which CK2 upregulation and Pml downregulation contribute to senescence evasion in Pten null tumours. Thus, in agreement with a model of intratumor heterogeneity, Pten loss promotes a senescence response that opposes tumour progression. However, a subset of Pten null cells upregulates CK2 that in turn promotes the evasion of cellular senescence by decreasing the level of Pml ( Supplementary Fig. 6i ). We believe that this mechanism may further contribute to the senescence evasion mediated by tumour-infiltrating myeloid cells in Pten null tumours [7] . Therefore, both cell autonomous and non-autonomous mechanisms can promote senescence evasion in tumours, suggesting that to design more efficient pro-senescence therapies for cancer, novel compounds should target both cell intrinsic and extrinsic factors. The existence of this novel PTEN–STAT3–CK2 network has also been validated in patients affected by prostate cancers through a bioinformatics analysis. Although we cannot rule out the possibility that additional genes may cooperate with PTEN loss to drive tumour progression, and demonstrate that the inhibition of CK2 is highly effective in blocking tumour development by enhancing senescence. Our results also indicate the need to monitor PTEN and CK2 status in clinical studies and highlight the importance of testing CK2 inhibitors alone or in combination with standard therapies in cancer patients. These drugs have acceptable toxicity profiles and are currently in clinical trials for different types of cancer [25] , [44] , [45] . In sum, our findings provide new insight into the mechanisms that regulate senescence evasion and encourage further efforts to screen for small molecules that could prove useful for pro-senescence therapy for cancer. Mouse crosses and MEF production Pten loxp/loxp mice were crossed with PB-Cre4 transgenic mice to generate prostate-specific deletion of Pten as previously reported [1] . MEFs were obtained by crossing male Pten loxp/loxp mice with female Pten loxp/loxp female. A pregnant mouse at 13 or 14 day post coitum was sacrificed by cervical dislocation. Embryos were harvested and the individual MEFs were cultured in DMEM containing 10% fetal bovine serum and 1% PenStrep. Primary Pten lox/lox MEFs were infected with retroviruses expressing either pMSCV-CRE-PURO-IRES-GFP or pMSCV-PURO-IRES-GFP for 48 h and selected with Puromycin at a concentration of 3 μg ml −1 and as previously described [1] . All mice were maintained under specific pathogen-free conditions in the animal facilities of the IRB institute, and the experiments were performed according to the state guidelines and approved by the local ethical committee. Human cancer cell lines Human prostate cancer cell lines ( Supplementary Table 3 ) were obtained from ATCC and were cultured according to manufacturer instructions. HCT116 isogenic cell line was a gift from Waldman lab. Pro-senescence screening platform The screening has been carried out in three steps. In the first step of the screening, compounds have been tested in triplicate in Pten −/− MEFs, plated in 96-well dishes, using a single drug concentration (10 μM). Compounds that promoted a strong growth arrest in Pten null MEFs (inhibition of proliferation ≥50%) have been considered positive hits and passed the first filter of the screening (efficacy filter). Positive hits were retested in triplicate at a single concentration (10 μM) in both Pten fl/fl and Pten −/− MEFs to assess growth arrest in both cell types (specificity filter). Compounds that pass the cell_specificity filter (inhibition of proliferation for Pten wt ≤20% and for Pten −/− ≥50%) were validated in duplicate in a dose–response assay in MEFs plated in 96-well dishes, to evaluate specificity at different concentrations (0.03–100 μM). Only the compounds having an optimal window of inhibition passed this filter (dose optimization filter). Finally, the compounds that passed all the filters were evaluated for SA-β-gal staining at three different concentrations in MEFs plated in 12-well dishes. Data shown refer to a single concentration (compound IC50). Data were normalized according to the negative control (dimethyl sulfoxide 100%). Nutlin-3, a previously characterized pro-senescence compound [26] was used as a positive control. Concentration response was analysed with XLfit (IDBS) by using four parameters logistic model. Proliferation and senescence assay Four days after treatment, MEFs were fixed for 20 min in a solution of buffered formalin (3.7%), washed with PBS (pH 7.3) and subsequently stained with a 0.01% crystal violet solution. After removing excess stain, the crystal violet stained cells were dissolved in 1 ml of 10% SDS solution overnight and the optical density of the extracted dye was read with a spectrophotometer at 590 nm. In the senescence assay, cells were stained for SA-β-gal activity, four days after treatment, using a senescence detection kit (Calbiochem). The number of blue stained cells were counted and normalized to the DAPI-positive cells. Generation of lentiviral shRNA kinome library An shRNA library in the pLKO.1 vector backbone comprising 3,280 shRNAs targeting 672 mouse kinases was obtained from Sigma. A pooled DNA preparation of the library was generated by growing bacterial cultures in deep-well 96-well plates inoculated from 96-well format bacterial glycerol stocks of the library. Culture medium was pooled and a midi-prep (Machery Nagel Nucleobond 500 kit) was performed to isolate plasmid DNA. Lentiviruses were produced by transfection of 293T cells with the pooled library DNA together with psPAX2 and pMD2G (gift from Didier Trono, EPFL Lausanne) and harvesting of culture supernatant between 48 and 72 h after transfection. Medium was filtered through a 0.45-μm filter and aliquots were frozen at −80 °C. Virus titre was determined by infecting NIH3T3 cells with serial dilutions of the virus and assaying colony formation in the presence of puromycin (4 μg ml −1 ). Kinome library screening Primary MEFs (5 × 10 6 ) derived from Pten fl/fl mice were cultured in an incubator maintained at 5% CO 2 and infected with the pooled mouse kinome lentiviral library at a multiplicity of infection of one functional viral particle per cell in the presence of polybrene (8 μg ml −1 ). Two days later, cells were split in three into medium containing puromycin (4 μg ml −1 ) alone to select for virally infected cells or puromycin together with Adenovirus expressing GFP (Vector Biolabs, 1060) or Cre-GFP (Vector Biolabs, 1700). Genomic DNA from the non-Adenovirus-infected cells after two further days of culture was isolated by incubation for 4 h with lysis buffer (200 mM NaCl, 50 mM Tris, 10 mM EDTA, 1% SDS) containing proteinase K (500 μg ml −1 ) and RNase A (83 μg ml −1 ) at 58 °C, followed by precipitation with NaCl/isopropanol and washing with 70% ethanol. The Adenovirus-infected cells were passaged every 3 days for a further 16 days before genomic DNA isolation. To maintain representation of the shRNA library in the population, at least 5 × 10 6 cells were utilized for genomic DNA isolation. To amplify the integrated shRNAs from the genomic DNA, PCR was conducted using a common forward primer containing sequencing adaptors and one of three reverse primers containing a barcode sequence specific for the experimental condition, as well as sequencing adapters. Forward primer 5′–3′ (bold highlights sequence of homology to pLKO.1): 5′-AATGATACGGCGACCACCGAGATCTACACTCTTTCCCTACACGACGCTCTTCCGATCTATCTTGTGGAAAGGACGA-3′ Reverse primers 5′–3′ (bold highlights Illumina Index six-nucleotide barcode sequences and sequence of homology to pLKO.1): 5′-CAAGCAGAAGACGGCATACGAGATATCACGGTGACTGGAGTTCAGACGTGTGCTCTTCCGATCTATTCTTTCCCCTGCACT-3′ 5′-CAAGCAGAAGACGGCATACGAGATTGGTCAGTGACTGGAGTTCAG ACGTGTGCTCTTCCGATCTATTCTTTCCCCTGCACT-3′ 5′-CAAGCAGAAGACGGCATACGAGATCACTGTGTGACTGGAGTTCAGACGTGTGCTCTTCCGATCTATTCTTTCCCCTGCACT-3′ Genomic DNA (15 ng) was used as PCR template in a 50-μl reaction containing 2.5 nmol of each primer, 5 U of Dream Taq (Thermo Scientific), 5 nmol dNTPs and 34 cycles at annealing temperature 56 °C and extension temperature 72 °C. The amplified PCR product was purified by excision from an agarose gel and purification using NucleoSpin Gel and PCR Clean-up kit (Macherey-Nagel) and subjected to 100 bp paired-end deep sequencing using an Illumina HiSeq 2000 machine. Bioinformatic analysis was used to identify each experiment using the unique barcodes and to map each individual sequencing read from the experiment to an individual hairpin sequence. For identification of experimental hits, shRNAs were first filtered for those represented by at least 200 reads at the early time point. Western blotting and histology Protein was isolated from whole MEFs cell pellets lysed with RIPA buffer and BCA protein assay reagent was used to determine the protein concentration. The following antibodies were used for western blotting: p21, p16, PAI-1 (Santa Cruz), CK2α, Pten, Hsp90 (Cell Signalling), PML (Millipore), p53 (Clone IMX25, Accurate Chemical Corp), pAKT Ser129 was produced in rabbit [30] , β-actin (Sigma) and E-cadherin (BD Biosciences). Secondary antibodies for mouse and rabbit were purchased from GE Healthcare. All dilutions are 1:1,000, except that β-actin antibody dilution is 1:5,000 and Secondary antibody dilution is 1:5,000. Full gel scans are shown in Supplementary Fig. 7 . For IHC and immunofluorescence, the tissues were embedded in 37% formaldehyde and embedded in paraffin for sectioning. CK2 shRNAs and PML siRNA transfection protocol Mouse CK2 pLKO shRNA vectors were obtained from Sigma. Using 293T HEKs, lentiviral particles were produced for negative control or shRNA vectors. MEFs were harvested after 72 h of infection for western blotting and SA-β-gal activity. shRNA sequences: 5′-CCGGACCTGTCAGCAGCGCCAATATCTCGAGATATTGGCGCTGCTGACAGGTTTTTTG-3′ (Clone ID:NM_007788.3-1293s21c1) and 5′-CCGGGCAATTGTACCAGACGTTAACCTCGAGGTTAACGTCTGGTACAATTGCTTTTTG-3′ (Clone ID:NM_007788.3-627s21c1). For the experiment with the PML siRNA, MEFs were transfected 1 day after selection using a smart pool PML siRNA (GE Healthcare, Dharmacon) and sequences of the siRNA targeting Pml from Qiagen used are 5′-CTGGATGTTCGATTCATGTAA-3′ and 5′-CCCAGCATATCTACTCCTTTA-3′. Luciferase reporter gene assay The promoter region of CSNK2A1 between −500 bp to +120 bp was cloned into a pGL4.24 luc2 vector to generate the CSNK2A1 reporter construct. Before transfection, immortalized MEFs were plated in 48-well plates and were co-transfected with CSNK2A1 reporter construct and a control pGL4.27 renilla TK vector in triplicates. The ratio of reporter to control plasmid was 10:1. After 48 h of transient transfection, cell lysates were transferred to 96-well plates and dual luminescence was measured using a Glo-Max Luminometer (Promega). Different CSNK2A1 mutants were generated by PCR mutagenesis. Primers used are shown in Supplementary Table 5 . Chromatin immunoprecipitation assay Immortalized MEFs were grown in T-75 flasks to a confluence of 90–95% and cells were fixed with 37% formaldehyde for 10 min and glycine for 5 min at room temperature. Nuclear extracts were sonicated using a Misonix 3,000 model sonicator to sheer crosslinked DNA to an average fragment size of ∼ 500 bp. Sonicated chromatin was incubated for 16 h at 4 °C with magnetic protein A beads (Millipore) conjugated with either anti-Stat3 antibody (Cell Signalling) or mouse IgG antibody (Millipore) by incubating overnight at 4 °C on a rotor. After incubation, beads were washed thoroughly and then centrifuged. The chromatin was eluted from the beads, and crosslinks were removed by incubation at 65 °C for 5 h. DNA was then purified using the QIAquick PCR Purification Kit (Qiagen). DNA was used to detect Stat3 binding to CK2 promoter sequences by qRT-PCR. The ChIP primers (5′-CAGCTGACAAACTGTAAAAGGGG-3′ and 5′-TGGGTTATTTCTGTACCAGCCATT-3′) were designed to amplify a region containing the putative Stat3-binding site (−1,228/−1,122 bp) in the mouse CK2 promoter As an internal negative control, the primers (5′-ATCCAGGATTATCAGGTTCAATTT-3′ and 5′-AGAGGTCTATGTCTGGGGGTGTAG-3′) were designed such that there is no putative Stat3-binding site (−2,184 to −2,083 bp). Primers pair used for positive control Socs3 are 5′-CCCTTGCAGTTCTAAGTTCAACA-3′ (forward) and 5′-ACCTTTGACAAGCGGACTCTC-3′ (reverse). Quantitative real-time PCR Quantitative real-time PCR was performed on RNA extracted from MEFs and prostatic tissues by using Trizol (Invitrogen) in triplicates. Complementary DNA was prepared with SuperScript III First-Strand Synthesis SuperMix (Invitrogen). Primers sequences used for p21, PAI-1, STAT3 and p16 are reported previously [42] and primers used for Pml forward 5′-CAGGCCCTAGAGCTGTCTAAG-3′, reverse 5′-ATACACTGGTACAGGGTGTGC-3′; Csnk2α forward 5′-AGGATAGCCAAGGTTCTGGGA-3′, reverse 5′-CCATCGCTTACGGGAGTGTC-3′; CSNK2α forward 5′-GGTGGAATGGGGAAATCAAGAT-3′, reverse 5′-TGATGATGTTGGGACCTCCTC-3′. Half-life determination and proteasome inhibitor MEFs were treated at 20 μg ml −1 concentration of cycloheximide and harvested at different time points for the analysis by western blotting. Proteosomal inhibitor MG132 was used at 10 μM in MEFs. PTEN and CK2 mRNA levels in human prostate cancer data sets Expression values for PTEN, CK2 and STAT3 were downloaded for Wallace [46] and Singh [47] prostate cancer data sets from Oncomine database [48] . Expression values for PTEN and CK2, as well as clinical information and follow-up was downloaded for Setlur [49] and Glinsky [50] data sets from Oncomine database. PTEN/CK2 mRNA ratio was calculated per each sample and patients were stratified into three groups by dividing the dataset into four percentiles (from highest to lowest value). Patients with lowest ratio values (1st percentile) were ascribed to group low (L), patients with intermediate values (2nd and 3rd percentiles) were ascribed to group intermediate (I) and patients with highest values (4th percentile) were ascribed to group high (H). Statistical analysis such as t -test, Pearson correlation and Kaplan–Meier curves were done using Stata 12.1 software. Differential expression of TFs Expression values for TFs in Pten pc+/+ normal prostates and Pten pc−/− tumours was downloaded from Gene Expression Omnibus database under the GSE24691 identifier, and the data have been previously reported [51] . t -test analysis was done to extract TFs with significant differential expression between mouse genotypes. Treatment with CK2 inhibitors CK2 inhibitors used were CK2i-Q quinalizarin (Sigma Aldrich), CK2i-CX (CX-4945 (Selleckchem)), K156 and K164 (ref. 15 ). CK2i-S (obtained in collaboration with Siena Biotech spa). CX-4945 sodium salt inhibitor administered in vivo treatment was synthesized by Shanghai Biochempartner Co. Ltd. Pten pc−/− mice at 8 weeks of age were treated by oral gavage with 75 mg kg −1 of CX-4945 or vehicle twice daily. CX-4945 was diluted in a solution with 25 mM NaH2PO4 buffer. After 4 weeks of treatment, prostate tumours were assessed for the size, number of PIN-affected gland and IHC. Functional annotation of targets and pro-senescence compounds All targets of the pro-senescence compounds were converted to HGNC compliant symbols and functionally annotated with experimentally biological processes comprised in gene ontology (GO; 14.10.2014) and Reactome (18.10.2014) using ClueGO 2.1.4 (ref. 52 ) and CluePedia 1.1.4 (ref. 52 ) within Cytoscape 3.1.1 (ref. 53 ). ClueGO analysis settings were set as follows: (i) Hierarchy levels=4 to 20, (ii) number of targets member of a biological process for the term to be mapped ≥1, (iii) percentage of a term covered by the targets ≥3%, (iv) GO-term fusion was applied and GO-term-grouping based on kappa score of 0.4 (similarity measure between the biological processes). For each group of terms and for terms that could not be grouped, the biological process that accommodated the largest number of targets was selected as overview term. All other settings were used as per default. Senescence pathways were extracted from a total of 25,517 gene sets (GSs) ( http://download.baderlab.org/EM_Genesets/May_14_2014/Human/symbol/Human_GO_AllPathways_with_GO_iea_May_14_2014_symbol.gmt ; 14.05.2014 and all curated GSs comprised in MSigDB v4.0 http://www.broadinstitute.org ) by filtering the GSs’ names for senescence and senescent . Any senescence pathway that had targets of a pro-senescence compound as members was mapped on the network. Thus, the network maps all pro-senescence compounds, the targets they inhibit, and the biological processes and senescence pathway. Statistical analysis Data analysis was performed using a two-tailed unpaired Student’s t -test. Data are represented as mean±s.d. How to cite this article: Kalathur, M. et al. A chemogenomic screening identifies CK2 as a target for pro-senescence therapy in PTEN-deficient tumours. Nat. Commun. 6:7227 doi: 10.1038/ncomms8227 (2015).